Ediacaran matground ecology persisted into the earliest Cambrian The beginning of the Cambrian was a time of marked biological and sedimentary changes, including the replacement of Proterozoic-style microbial matgrounds by Phanerozoic-style bioturbated mixgrounds. Here we show that Ediacaran-style matground-based ecology persisted into the earliest Cambrian. Our study in the type section of the basal Cambrian in Fortune Head, Newfoundland, Canada reveals widespread microbially induced sedimentary structures and typical Ediacaran-type matground ichnofossils. Ediacara-type body fossils are present immediately below the top of the Ediacaran but are strikingly absent from the overlying Cambrian succession, despite optimal conditions for their preservation, and instead the microbial surfaces are marked by the appearance of the first abundant arthropod scratch marks in Earth evolution. These features imply that the disappearance of the Ediacara biota represents an abrupt evolutionary event that corresponded with the appearance of novel bilaterian clades, rather than a fading away owing to the gradual elimination of conditions appropriate for Ediacaran preservation. The Agronomic Revolution (and the related concept of the Cambrian Substrate Revolution) marks the replacement of matgrounds by bioturbated mixgrounds, in an event that had profound palaeoecological, evolutionary and taphonomic consequences [1] , [2] , [3] . This event is thought to have taken place at the beginning of the Phanerozoic, signalling the establishment of modern-style ecosystems after 3 billion years of mostly microbial evolution [4] . On the basis of detailed analysis of the type section of the Fortunian (lowermost Cambrian) at the Global Stratotype (GSSP) for the Cambrian System in Fortune Head, southeast Newfoundland, Canada [5] , [6] , we document widespread microbially induced sedimentary structures (MISSs [7] ) and associated trace fossils, indicating that a microbial matground-based ecology actually persisted well into the early Cambrian. This study has significant implications with respect to the evolutionary history of the Ediacara biota because it shows a continuity of the Ediacaran taphonomic window into the early Cambrian, implying that the disappearance of this biota cannot be attributed solely to the lack of adequate preservational conditions [8] . Stratigraphical and palaeoenvironmental setting Basal Fortunian strata in Burin Peninsula of southeast Newfoundland are represented by Member 2 of the Chapel Island Formation [5] . These deposits dominantly record sedimentation in shallow marine and deltaic settings under storm influence, as indicated by the abundance of combined-flow and wave-generated sedimentary structures, such as symmetrical to quasi-symmetrical ripples, and hummocky cross-stratification, graded tempestites, and pot and gutter casts [9] , [10] , [11] , [12] . A variety of soft-sediment deformation structures and mass-flow deposits reflect prodeltaic deposition [13] . MISS MISS and associated biogenic structures are abundant throughout Member 2. Wrinkle marks are the dominant structures ( Fig. 1a–c ), and small gas domes occur as well ( Fig. 1d ), both at the top of very fine-grained silty sandstone. A detailed survey of bedding planes indicates that ~75% of the surfaces in the studied sections contain MISS. Of the bedding planes containing MISS, 10–50% of the exposed surface is covered with MISS. Wrinkle marks are characterized by small, subparallel, slightly curved, relatively continuous crests and troughs. Most authors agreed that these structures form while the sediment is biostabilized by microorganisms; some considered them as preserved surfaces with microbial mats [14] , whereas others interpreted wrinkle structures as formed beneath the mats [15] . Most of these wrinkles are associated with superbly preserved, delicate, horizontal trace fossils. Small gas domes consist of subspherical protrusions on bedding planes. They form owing to the accumulation of gases derived from different sources, such as organic matter decay and oxygen produced during photosynthesis. These gases are trapped beneath the impermeable mat layer, forming an upward bulge on the sedimentary surface [16] , [17] . The size of gas domes is in direct proportion to the thickness of the microbial mat [16] . In the present case, gas domes are relatively small (that is, <1 cm wide), suggesting a thin microbial mat or biofilm. Analysis of thin sections reveals the presence of continuous layers of microbial mats. Large quantities of pyrite, typically oriented parallel to the palaeosurface, occur close to the mat layers. The presence of pyrite in close association with the mat layers suggests reducing chemical conditions beneath the mats. Further evidence of a microbial mat origin for these structures is provided by the associated trace fossils. Most of the beds with MISS have trace fossils preserved not only as negative epireliefs but also as positive epireliefs, which is the typical preservation style of biogenic structures formed slightly below biofilms [8] . Also, the superb preservation of Allocotichnus ( Fig. 1e ) as delicate negative impressions on an upper bedding surface is allowed by the presence of microbial mats, because preservation of fine morphologic details is especially favoured in microbially stabilized substrates [18] . In short, the available evidence (for example, wrinkle structures and gas domes, presence of pyrite and floating grains in close association with the wrinkled surfaces and excellent preservation of delicate trace fossils) collectively support our interpretation of the presence of extensive microbial mats on these Fortunian surfaces. 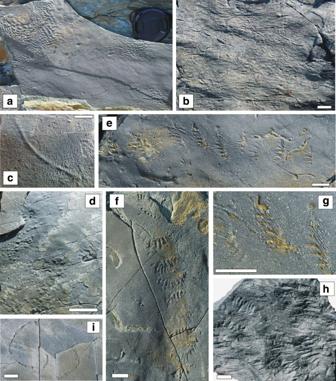Figure 1: Microbially induced sedimentary structures and trace fossils in Member 2 of the Chapel Island Formation. All images are of upper bedding surfaces. (a) Patches of wrinkle marks andCochlichnus anguineus. Lens cap diameter is 5.5 cm. (b) Poorly preserved wrinkle marks covered with grazing trails, namelyCochlichnus anguineusandHelminthopsis tenuis. Scale bar, 1 cm. (c) Close-up ofHelminthoidichnites tenuisassociated with wrinkle marks. Scale bar, 1 cm. (d) Small gas domes and tinyHelminthoidichnites tenuis. Scale bar, 1 cm. (e) Specimen ofAllocotichnus dyeri. Scale bar, 1 cm. (f) Specimen ofAllocotichnus dyeri. Note associatedHelminthoidichnites tenuis. Scale bar, 1 cm. (g) Close-up of the specimen ofAllocotichnus dyeriillustrated ine, showing preservation of delicate morphologic details. Scale bar, 1 cm. (h) Negative epirelief preservation of the trilobite resting traceRusophycus avalonenesis. Scale bar, 1 cm. (i)Treptichnus coronatum. Scale bar, 1 cm. Figure 1: Microbially induced sedimentary structures and trace fossils in Member 2 of the Chapel Island Formation. All images are of upper bedding surfaces. ( a ) Patches of wrinkle marks and Cochlichnus anguineus . Lens cap diameter is 5.5 cm. ( b ) Poorly preserved wrinkle marks covered with grazing trails, namely Cochlichnus anguineus and Helminthopsis tenuis . Scale bar, 1 cm. ( c ) Close-up of Helminthoidichnites tenuis associated with wrinkle marks. Scale bar, 1 cm. ( d ) Small gas domes and tiny Helminthoidichnites tenuis . Scale bar, 1 cm. ( e ) Specimen of Allocotichnus dyeri . Scale bar, 1 cm. ( f ) Specimen of Allocotichnus dyeri . Note associated Helminthoidichnites tenuis . Scale bar, 1 cm. ( g ) Close-up of the specimen of Allocotichnus dyeri illustrated in e , showing preservation of delicate morphologic details. Scale bar, 1 cm. ( h ) Negative epirelief preservation of the trilobite resting trace Rusophycus avalonenesis . Scale bar, 1 cm. ( i ) Treptichnus coronatum . Scale bar, 1 cm. Full size image Matgrounds and trace fossils A wide variety of trace fossils occur in direct association with the MISS at the top of sandstone beds typically covered by a thin veneer of siltstone. The trace fossils are restricted to bedding planes, typically cross-cut wrinkle marks, and do not produce significant disruption of the primary sedimentary fabric. Analysis of the matground facies shows three main types of trace fossils. First, grazing trails, namely Cochlichnus anguineus ( Fig. 1a,b ), Helminthopsis tenuis ( Fig. 1b ) and Helminthoidichnites tenuis ( Fig. 1c,d ), are preserved either as negative or positive epireliefs, and record grazing of organic matter concentrated within microbial mats below a thin veneer of sediment ( Helminthopsis ichnoguild). Second, trackways and various scratch marks, attributed to Allocotichnus dyeri ( Fig. 1e–g ) and Diplichnites isp., as well as the resting trace Rusophycus avalonensis ( Fig. 1h ), are typically preserved as negative epireliefs and were produced by arthropods scratching the surface of the mat ( Diplichnites ichnoguild). The presence of tiny scratch marks, showing delicate morphologic details, superbly preserved on upper bedding surfaces, implies considerable substrate consistency as would have been expected in a rigid microbial mat. The third type of structure consists of three-dimensional branching burrows, namely Treptichnus pedum , T. coronatum ( Fig. 1i ) and T. pollardi . These full-relief branching structures were emplaced slightly below the mat surface, and therefore are regarded as produced by undermat miners ( Treptichnus–Saerichnites ichnoguild), most likely worm-like organisms, such as priapulids [19] . After the Agronomic Revolution, matgrounds retreated to stressful environments in which bioturbation was mostly inhibited, such as dysoxic shelves or tidal flats affected by subaerial exposure and salinity fluctuations [14] , [15] , [20] , [21] , [22] . The extensive occurrence of matground and associated trace fossils in the Fortunian outcrops of Fortune Head indicates that the quintessential Ediacaran-style ecology persisted into the Phanerozoic. These microbial matground-dominated ecosystems can be regarded as relict Ediacaran ecosystems because the sediment was dominated by microbially bound surfaces that were exploited by benthic communities. This is consistent with evidence from roughly coeval deposits in China from which structures indicative of animal–matground interactions are common, including radular marks and possible undermat mining burrows, further supporting our view of relict Ediacaran strategies persisting in the early Cambrian [23] . Microbial stabilization probably played some role until later in the Cambrian, as suggested by the abundance of echinoderm faunas dominated by shallow sediment stickers and sediment attachers [24] . However, the evolutionary innovations of the Cambrian explosion allowed for more complex interactions to develop, making the Fortunian a pivotal point in the history of the biosphere [25] , [26] . This combination of a microbial matground-based ecology and the appearance of new body plans and associated locomotory mechanism, actually resulted in a peak in diversity of animal–matground interactions during the Fortunian ( Fig. 2 ). The grazing trace fossils are essentially identical to those from the Ediacaran matgrounds [25] , [27] , revealing continuity across the Ediacaran–Cambrian boundary of microbial grazing as one of the most widespread feeding strategies. The appendage imprints reflect the appearance of a new cast of matground scratchers. During the Ediacaran, this strategy was represented by a probable stem-group mollusk Kimberella and associated scratch marks ( Kimberichnus ) produced by its paired radular teeth on microbial surfaces [28] , [29] , [30] , [31] . Recent claims that the scratch marks represent ice needles [32] are unsubstantiated, and fail to explain their direct association with Kimberella . During the Fortunian, the appearance of arthropods is signalled by the presence on matgrounds of superbly preserved trackways and scratch marks, revealing rasping of the microbial surfaces. In any case, arthropods had not yet assumed the role of major bioturbators that they filled later in the Phanerozoic. The three-dimensional burrows represent a novel way of interacting with the matgrounds because systematic undermat mining structures are virtually unknown in Ediacaran strata. In the Fortunian, this strategy is recorded by the appearance of systematically branching burrow systems exploiting the organic matter concentrated within microbial mats from below. In Fortunian rocks in Newfoundland and elsewhere, sophisticated strategies involving strophotaxis (proclivity to make U-turns so that the animal turns around 180° at intervals), phobotaxis (which prevents the organism from crossing its own and other trails) or thigmotaxis (which makes the animal to keep close contact with a former trail) have been documented in microbial matgrounds by the presence of ichnospecies of Oldhamia , which reveal complex morphological patterns [26] , [29] , [33] . Direct external digestion of the mat, which has been suggested for the Ediacaran Dickinsonia [34] and represented by the ichnogenus Epibaion [31] , is a type of animal–matground interaction unrecorded in the Cambrian. 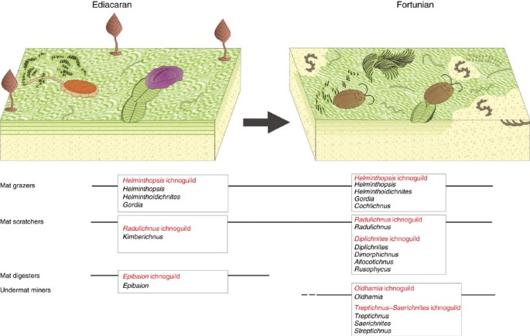Figure 2: The ichnological record of animal–matground interactions across the Ediacaran–Fortunian transition. Some types of interactions are restricted to the Ediacaran (mat digestion), whereas others cross the Ediacaran–Fortunian essentially unaffected (mat grazers), display significant compositional changes (mat scratching), or represent Fortunian innovations (undermat mining). Although Ediacaran grazing trails associated with matgrounds have been commonly regarded as undermat miners, they do not represent construction of branching feeding tunnels (feeding structures or Fodinichnia) and they should be regarded as mat grazers (grazing traces or Pascichnia). Cambrian radular scratch marks are provisionally included inRadulichnus, pending more detailed analysis. Figure 2: The ichnological record of animal–matground interactions across the Ediacaran–Fortunian transition. Some types of interactions are restricted to the Ediacaran (mat digestion), whereas others cross the Ediacaran–Fortunian essentially unaffected (mat grazers), display significant compositional changes (mat scratching), or represent Fortunian innovations (undermat mining). Although Ediacaran grazing trails associated with matgrounds have been commonly regarded as undermat miners, they do not represent construction of branching feeding tunnels (feeding structures or Fodinichnia) and they should be regarded as mat grazers (grazing traces or Pascichnia). Cambrian radular scratch marks are provisionally included in Radulichnus , pending more detailed analysis. Full size image The fact that the Fortunian represents a transition point in animal–substrate interactions is further demonstrated by the presence of more intensely bioturbated siltstone, which is interbedded with the matground facies. Typically, the preserved microbial mats occur on the top of sandy event beds, indicating minor omission surfaces. Re-establishment of background fair-weather sedimentation was apparently associated with more thorough bioturbation, reflecting the alternation of both types of ecologies within the same depositional environment. However, this fair-weather bioturbation cannot be regarded as of Phanerozoic-style because instead of poorly defined mottled textures, such as those formed in the modern mixed layer, it consists of well-defined biogenic structures with clear burrow boundaries. This is indicative of firmground conditions close or at the sediment surface [35] , [36] . Most of the Ediacaran succession exposed at the GSSP consists of intertidal deposits [9] , [12] , an environmental setting that was not conducive to the Ediacara biota [37] , [38] . Palaeopaschichnus, a soft-bodied fossil restricted to Ediacaran strata worldwide [39] , occurs in subtidal strata 0.2 m below the top of the Ediacaran at the GSSP [5] , but despite intensive search no Ediacara-type body fossils have been found in the overlying Cambrian succession. The disappearance of the Ediacara biota, and its replacement by a fauna of complex metazoans is still a puzzling issue, and three alternative hypotheses have been invoked: mass extinction of Ediacaran forms; biotic replacement, either as a result of predatory displacement or ecosystem engineering; and closing of the unique Ediacaran taphonomic window [40] . The persistence of widespread MISS and associated trace fossils indicative of a wide variety of interactions between bilaterians and microbial matgrounds throughout the whole of Member 2 of the Chapel Island Formation suggests that the typical Ediacaran taphonomic window [41] persisted during ~10 million years into the Phanerozoic. Simple non-diagnostic discs, vaguely similar to those present in the Ediacaran, have been locally recorded in lower Cambrian outcrops elsewhere [23] as have other enigmatic remains [42] , [43] . However, no representatives of iconic members of the Ediacara biota, such as Dickinsonia , Kimberella , Tribrachidium or Palaeopaschichnus are preserved in these deposits, despite the presence of appropriate sedimentary facies and preservational conditions. Our study indicates that the disappearance of the Ediacara biota cannot be attributed to the elimination of unique taphonomic conditions (that is, the Cheshire Cat model [40] ). In addition, the loss in disparity and diversity of the Ediacara biota some 5 million years before the Ediacaran–Cambrian transition further argues against the Cheshire Cat model and a mass extinction hypothesis, suggesting instead a more gradual extinction [40] . In the same vein, the continuity of the matground taphonomic window across the Ediacaran–Cambrian boundary indicates that the well-known absence of arthropod-generated structures in Ediacaran matgrounds [18] cannot be attributed to a lack of appropriate preservational conditions and that their appearance immediately above the basal Cambrian boundary at Fortune Head represents evolution rather than taphonomy. Collectively, these data imply that the disappearance of the Ediacara biota, and the appearance of arthropods capable of making scratching traces, represent true evolutionary events that were nearly coincident with the Ediacaran–Cambrian boundary. Integration of the available palaeontological, ichnological and sedimentological information is consistent with the notion that the Ediacara biota was outcompeted by new bilaterian clades that mark the dawn of the Phanerozoic. Sedimentological and ichnological analysis This paper is based on an integrated detailed sedimentological and ichnological study of 19 bedding surfaces containing MISS, combining both field observations and thin-section analysis. Standard facies analysis includes characterization of lithology, physical sedimentary structures, contact and geometry of the intervals containing MISS. Ichnological analysis involves limited trace fossil sampling, recognition and identification of the ichnofossils present; study of density, abundance and distribution of individual ichnotaxa; identification of trophic types and ethologic groups; and relationships among trace fossils and MISS in each bed. Field collections Because field work took place in the Fortune Head Ecological Reserve (under a Scientific Research Permit from Parks and Natural Areas, Newfoundland and Labrador), sampling was kept to a minimum and oriented to thin-section analysis with the aim of establishing details of trace fossils and MISS relationships. Outcrop location A location map of the outcrops studied is provided in Supplementary Fig. 1 . The outcrops studied are illustrated in Supplementary Fig. 2 . Sedimentological logs of Member 2 of the Chapel Island Formation have been presented elsewhere [5] , [9] , [10] , [11] , [12] , [13] . Detailed sections of two selected intervals containing MISS are provided in Supplementary Fig. 3 . Additional field photos of relevant structures are presented in Supplementary Figs 4–7 , whereas a thin-section photograph of MISS is provided in Supplementary Fig. 8 . How to cite this article: Buatois, L. A. et al. Ediacaran matground ecology persisted into the earliest Cambrian. Nat. Commun. 5:3544 doi: 10.1038/ncomms4544 (2014).